A shared genetic basis of mimicry across swallowtail butterflies points to ancestral co-option ofdoublesex Uncovering whether convergent adaptations share a genetic basis is consequential for understanding the evolution of phenotypic diversity. This information can help us understand the extent to which shared ancestry or independent evolution shape adaptive phenotypes. In this study, we first ask whether the same genes underlie polymorphic mimicry in Papilio swallowtail butterflies. By comparing signatures of genetic variation between polymorphic and monomorphic species, we then investigate how ancestral variation, hybridization, and independent evolution contributed to wing pattern diversity in this group. We report that a single gene, doublesex (dsx) , controls mimicry across multiple taxa, but with species-specific patterns of genetic differentiation and linkage disequilibrium. In contrast to widespread examples of phenotypic evolution driven by introgression, our analyses reveal distinct mimicry alleles. We conclude that mimicry evolution in this group was likely facilitated by ancestral polymorphism resulting from early co-option of dsx as a mimicry locus, and that evolutionary turnover of dsx alleles may underlie the wing pattern diversity of extant polymorphic and monomorphic lineages. An array of convergent adaptations are found across animal and plant taxa, arising from the interplay of natural selection, constraint, and historical contingency [1] . Comparing the genetic basis of convergent traits has been central to uncovering the genomic patterns and evolutionary processes that drive adaptation and phenotypic diversification [2] . By leveraging natural experiments of convergent adaptation, we are able to assess the extent to which evolution proceeds with shared genetic architecture, genes, and/or mutations. Furthermore, comparing how these evolutionary changes unfold in the genome among multiple taxa can uncover how ancestral variation, hybridization, or independent evolutionary trajectories contribute to adaptive phenotypes [3] . Mimicry is a major convergent adaptation, and a significant driver of phenotypic evolution across animals and plants [4] . Much of our knowledge about the molecular foundations and evolution of mimicry has stemmed from research on wing pattern mimicry in butterflies [5] , [6] , [7] , [8] , [9] , [10] , [11] , a fundamental adaptation known to involve a diverse set of genes and genetic architectures. Perhaps the most extreme version of this adaptation is found in polymorphic mimicry, where discrete mimetic phenotypes co-occur within a species. Polymorphic mimicry has evolved in multiple butterfly lineages [9] , [12] , [13] , providing an opportunity to investigate the genetics and evolutionary origins of this complex adaptation. In Heliconius numata , polymorphic mimicry is controlled by a cluster of wing patterning genes contained within a chromosomal inversion [9] , [14] . This mimicry supergene along with other mimicry alleles are the product of frequent introgressive hybridization in the Heliconius clade [10] , [14] . In the genus Papilio , where polymorphic mimicry is typically limited to females, several independent molecular origins have been implicated in the evolution of wing pattern mimicry. Classic genetic crossing experiments on various Papilio species showed that either sex-linked or autosomal loci can function as ‘switches’ between female morphs [5] , [6] , [8] , and more recent molecular work has identified and characterized some of these mimicry loci [11] , [15] , [16] , [17] . In each of these studies, the mimicry loci of different Papilio species are located in distinct regions of the genome, with seemingly independent functional bases. These single-species analyses have illustrated the diverse molecular underpinnings generating polymorphic wing patterns. However, a comparative analysis of multiple polymorphic and monomorphic lineages is needed to elucidate the relative contributions of historical contingency and contemporary allele sharing to the evolution of mimicry and wing pattern diversity in this group. Polymorphic mimicry is inferred to have evolved independently in several Papilio lineages [12] , [13] , but questions remain about the potential roles of ancestral variation and contemporary allele sharing in shaping the extant diversity of Papilio wing pattern phenotypes. Multiple Papilio species are known to share mimicry supergene architecture [5] , [7] , [8] , in which wing pattern variation is transmitted as a single Mendelian locus. More recently, studies in both P. polytes and P. memnon characterized their mimicry loci as having the same identity, the autosomal gene doublesex ( dsx ) [11] , [17] , [18] , [19] . The dsx mimicry alleles are distinct between P. polytes and P. memnon [18] , [19] , but without knowledge of dsx variation among other closely related species it is uncertain whether dsx -mediated mimicry arose de novo or as a product of shared ancestral variation. The extent to which dsx mediates polymorphic mimicry in other Papilio lineages, and how variation at dsx is related between polymorphic and monomorphic lineages are thus open questions that are pivotal to understanding the roles of genetic potentiation, constraint, and shared ancestry in mimicry evolution. In this study, we test for convergence in the genetic basis of mimicry among four closely related female polymorphic lineages, P. polytes , P. memnon , P. rumanzovia , and P. aegeus . We test whether the evolution of polymorphic mimicry involves changes at the same genomic location, and we find that the same gene, dsx , controls female polymorphic mimicry in all four species. We then analyze closely related monomorphic lineages to infer the historical processes driving mimicry evolution and wing pattern diversity across this group. Specifically, we explore four hypotheses for the evolution of mimicry in this clade: (1) introgression, (2) ancestral polymorphism with incomplete lineage sorting, (3) ancestral polymorphism with allelic turnover, and (4) independent evolution (Fig. 1 ). In (1), mimicry alleles are transmitted between hybridizing lineages by introgression (Fig. 1a ). In (2), polymorphic mimicry evolves ancestrally and the ancestral mimicry alleles are inherited and maintained by multiple lineages through balancing selection (Fig. 1b ). In (3), polymorphic mimicry evolves ancestrally, but mimicry alleles are subsequently replaced by their own allelic descendants, or lost by drift, a process known as allelic turnover [20] , [21] , [22] (Fig. 1c ). In (4), mimicry alleles arise independently in each lineage by repeated co-option of dsx (Fig. 1d ). Our results indicate the presence of distinct dsx mimicry alleles among species, ruling out both introgression and incomplete lineage sorting. While we cannot rule out the possibility of independent dsx co-option, we do find evidence consistent with allelic turnover. Independent evolution and allelic turnover are expected to result in distinct alleles among species, but allelic turnover will produce allelic genealogies with elongated branches due to underlying multiallelic balancing selection [22] , [23] . Similarly, population genetic signatures associated with balancing selection can be used to differentiate independent evolution from allelic turnover. Together with previous work, our findings suggest that ongoing turnover of dsx alleles from a polymorphic ancestor underlies much of the wing pattern diversity in this group. These findings imply a dynamic trajectory for mimicry evolution, potentially involving many gains and losses of mimicry alleles. Fig. 1: True (top row) and inferred (bottom row) genealogies under four mimicry evolution hypotheses. Colors represent distinct mimicry alleles/phenotypes. a Mimicry alleles are shared because of introgressive hybridization. b Mimicry evolves ancestrally, and descendant lineages inherit and maintain the ancestral alleles. c Mimicry evolves ancestrally, and alleles are gained and lost so that the extant alleles are distinct from the ancestral alleles. d Unique mimicry alleles arise by the independent evolution of mimicry. Under introgression and incomplete lineage sorting (ILS), the inferred genealogies will show alleles grouping by phenotype rather than species ( a , b ), but the branch lengths will be relatively shorter for introgression than for ILS. Under allelic turnover and independent evolution, the inferred genealogies will result in alleles grouping by species ( c , d ), but the branch lengths are expected to be longer for allelic turnover because of underlying balancing selection. A history of allelic turnover will also leave behind population genetic signatures of balancing selection, such as elevated Tajima’s D in the region of interest. Under allelic turnover, the amount of shared ancestral variation should track phylogenetic relatedness, because recombination and gene conversion will erase the evidence of ancestral variants as a lineage ages. Because shared ancestral variation is more likely to be retained at younger timescales, allelic genealogies may show alleles of one species nested within another species for younger lineages. In contrast, independent evolution need not involve balancing selection, and if variants are shared among lineages, these should not be correlated with the lineages’ phylogenetic proximity. Full size image Mimicry loci in P. rumanzovia , P. memnon , P. aegeus We first identified the mimicry loci of P. rumanzovia , P. memnon , and P. aegeus using genome-wide association studies (GWAS) and principal component analyses (PCA) of single nucleotide polymorphism (SNP) data. We analyzed female specimens representing three P. rumanzovia morphs (simple, blended, white), two P. memnon morphs (band, patch), and two P. aegeus morphs (light, dark). In P. rumanzovia , a GWAS with the three morphs and 869,047 variants revealed a single peak of association positioned within the dsx gene (Fig. 2a ). In additional GWAS comparing pairs of morphs we observed the same peak of variants in the dsx region for the simple/white and blended/white comparisons, but not for the simple/blended (Supplementary Fig. 1 ). For the simple/blended GWAS, only one highly associated variant remained within the dsx region, and several emerged in the vicinity of dsx (Supplementary Fig. 1C ). We next sought to characterize the population substructure associated with dsx mimicry alleles using methods originally developed to identify chromosomal inversions from SNP data [24] . We compared population structure to local dsx genotypes using principal component analysis (PCA) based on genome-wide SNPs and PCA based on dsx SNPs. The genome-wide PCA based on ~2.5 million SNPs placed most individuals into a single cluster (Fig. 2b ). In contrast, the dsx PCA for the same individuals based on 779 dsx -specific SNPs resulted in the white individuals separating from the simple and blended individuals along PC1 (Fig. 2c ). Most of the white individuals were found to be heterozygous at dsx , resulting in their intermediate placement along PC1 (Fig. 2c ). These results suggest that variation at the dsx locus differentiates the P. rumanzovia white patch morph from the simple and blended morphs, and that the simple and blended morphs may be determined by variation in and around dsx . Fig. 2: Identifying mimicry loci in P. rumanzovia , P. memnon , and P. aegeus . Genome-wide association study (GWAS) for wing patterning in P. rumanzovia ( a ) and P. memnon ( d ). Principal component analysis (PCA) based on genome-wide variants for P. rumanzovia ( b ), P. memnon ( e ), and P. aegeus ( g ). PCA based on dsx variants for P. rumanzovia ( c ), P. memnon ( f ), and P. aegeus ( h ). Red points in a and d indicate SNPs in the dsx region. Dashed and dotted lines in a and d show the false discovery rate ( q -value) cutoffs of 0.01 and 0.001, respectively. Full size image The GWAS for P. memnon using approximately 1.8 million variants showed noise in genome-wide association values, but the densest cluster of highly associated variants fell within the dsx region (Fig. 2d ). The genome-wide PCA (~2.5 million SNPs) revealed that white band morphs differ from white patch morphs across the genome, possibly due to different geographic origins of our band and patch samples. This causes variants across the genome to appear highly associated with wing pattern phenotype (Fig. 2d ), when in reality these variants are unrelated to wing patterning. The PCA for the same set of individuals based on 644 dsx -specific SNPs segregated individuals by wing pattern along PC1 (Fig. 2f ). These results point to dsx as the mimicry locus in P. memnon , consistent with other recent works on P. memnon [18] , [19] . We were not able to generate GWAS results for P. aegeus due to low sample size. The PCA for approximately 1.5 million genome-wide SNPs revealed differentiation between light and dark morphs across the genome, as in P. memnon (Fig. 2g ), but the PCA with only dsx SNPs (500 SNPs) showed individuals segregating by phenotype along PC1 (Fig. 2h ). Like in P. rumanzovia , the light morph individuals were nearly all dsx heterozygotes and fell in the center of PC1 (Fig. 2h ). From these results, we concluded that dsx is also associated with polymorphic wing patterning in P. aegeus . Genetic differentiation and linkage disequilibrium at dsx We calculated F ST between wing pattern morphs within each polymorphic species to analyze patterns of genetic differentiation across the mimicry locus dsx . For each comparison, we applied a 10 kb window size across the genome and removed windows with a low number of variants (bottom 10% by species). We visualized the genetic differentiation between morphs across the dsx region and compared these values to the genome-wide F ST distribution. First, we calculated F ST between the mimetic and non-mimetic P. polytes female morphs as a positive control for highly divergent, inverted dsx haplotypes [11] , [17] . We observed a plateau of elevated F ST across the entire dsx region, reflecting the inverted chromosomal structure of dsx in P. polytes (Fig. 3a ). Furthermore, the highest F ST value for dsx windows was in the 99th percentile of the genome-wide distribution of F ST values (Fig. 3b ). In subsequent comparisons for P. rumanzovia , P. memnon , and P. aegeus , each species showed elevated F ST at dsx relative to the rest of the genome, but we observed species-specific patterns of differentiation within the dsx region. For P. rumanzovia , we calculated F ST between the three pairs of morphs (simple/white, blended/white, simple/blended) using the 23 individuals from the PCAs. The results showed high F ST for dsx windows in comparisons between simple/white and blended/white, consistent with the GWAS and PCA results, but this region of elevated F ST did not include exon one (Fig. 3g, i ). The highest F ST value for dsx windows in each of the simple/white and blended/white comparisons was also in the 99th percentile of their respective genome-wide F ST distributions (Fig. 3h, j ). Between the simple and blended morphs, only one dsx window showed elevated F ST , driven by the single highly associated SNP we observed in the GWAS (Fig. 3k , Supplementary Fig. 1C ). In P. memnon , the entire length of dsx showed elevated F ST between the 20 band individuals and 9 patch individuals, resembling the plateau observed across dsx in P. polytes (Fig. 3c ). For P. aegeus , the elevated dsx F ST was restricted to the window containing exon one and the window containing exon four (Fig. 3e ). The highest F ST value for dsx in both P. memnon and P. aegeus was in the 99 th percentile of their respective genome-wide distributions, consistent with earlier GWAS and PCA (Fig. 3d, f ). Fig. 3: Genetic differentiation between morphs. F ST across a 500 kb interval containing dsx (gray box) in P. polytes ( a ), P. memnon ( c ), P. aegeus ( e ), and P. rumanzovia ( g , i , k ). E1–6 indicate the position of dsx exons. Genome-wide F ST distribution in P. polytes ( b ), P. memnon ( d ), P. aegeus ( f ), and P. rumanzovia ( h , j , l ). Red arrows indicate the highest F ST value for dsx windows, all of which are in the 99th percentile of their respective distributions. Full size image We next analyzed patterns of linkage disequilibrium (LD) within dsx and the surrounding region for each species, again using P. polytes as a positive control for highly differentiated mimicry haplotypes. P. polytes showed high LD across the entire length of dsx , consistent with prior analyses and the known inversion spanning the dsx region [17] (Fig. 4a ). In P. rumanzovia , a subset of the dsx region spanning exons two through six showed elevated LD, reflecting the region of elevated F ST described above (Figs. 4b , 3g, i ). For P. memnon we observed a region of elevated LD across the length of dsx like in P. polytes , corroborating the high F ST plateau across this region (Figs. 4c , 3c ). The elevated LD signature for dsx in P. aegeus was localized to a region containing exon one, which was also consistent with the F ST results (Figs. 4d , 3e ). Fig. 4: Linkage disequilibrium (LD) heat maps. LD across dsx (gray shading) and flanking 100 kb for P. polytes ( a ), P. rumanzovia ( b ), P. memnon ( c ), and P. aegeus ( d ). Standard color scheme: D’ < 1, LOD < 2 (white); D’ = 1, LOD < 2 (blue); D’ ≤ 1, LOD ≥ 2 (pink and red). Dashed line in a shows the inverted region. E1–6 indicate the dsx exons. Full size image De novo genome assembly in P. rumanzovia We generated de novo genome assemblies for P. rumanzovia to validate our methods and explore structural variation at dsx . We used combined mate-pair and paired-end sequencing datasets to assemble the genomes of one female that we inferred to be homozygous for the simple morph-associated haplotype and one female inferred to be homozygous for the white morph-associated haplotype. The assembled genome sizes for the simple and white morph were 218 and 215 Mb, respectively, which are similar to the 227 Mb P. polytes genome [11] , [17] . The scaffold N50 values for the simple and white assemblies were 53 kb and 197 kb, respectively. We identified four scaffolds in the simple morph assembly and three scaffolds in the white morph assembly that contained dsx exons (Supplementary Fig. 2 ). In the simple morph assembly, two scaffolds provided structural information. First, exons two through four were assembled on a single scaffold, at approximately the same distance and orientation to one another as in P. polytes . Second, exon six and the neighboring ubiquitously expressed transcript (UXT) were assembled together, revealing the collinearity of the simple morph with the non-mimetic P. polytes morph and with the outgroup taxon P. xuthus . With the white morph assembly, we could gather structural information from one scaffold which contained exons one through four arranged at approximately the same distance and orientation as in P. polytes . Our comparisons of the simple and white morph showed a sharp increase in F ST and LD between exons one and two, and a drop in these signatures between exons five and six (Figs. 3 g, 4b ), which could be indicative of a chromosomal inversion in this region. This inversion would have to be in the simple morph, given that exons one through four coassembled onto a single  white morph scaffold. Together, these data show that if there exists a dsx inversion in P. rumanzovia , its breakpoints are quite different from those of P. polytes . We aligned the scaffolds containing dsx exons to further explore sequence differentiation between the P. rumanzovia simple and white morphs (Supplementary Fig. 2 ). Consistent with the F ST analysis (Fig. 3g ), we generally observed higher sequence identity surrounding exon one and much lower identity for regions surrounding exons two through six. In contrast to the numerous substitutions between the P. polytes mimetic and non-mimetic across exons one through six, we found that the simple and white P. rumanzovia sequences differed only at exons five and six, and had identical sequences for exons one through four. Exon five, however, is only spliced into the male dsx isoform in P. polytes , and exon six is a non-coding exon [11] . While we cannot conclude what the functional impacts of these differences are, these results appear to indicate that the switching between female mimicry phenotypes in P. rumanzovia is not a result of dsx protein coding differences, but likely a regulatory phenomenon. Evolutionary relationships between dsx haplotypes In order to trace the evolutionary history of dsx -mediated wing pattern polymorphism we characterized the phylogenetic relationships of polymorphic and monomorphic Papilio species using both genome-wide SNPs and phased dsx SNPs. We generated a maximum-likelihood species tree based on ~3.4 million SNPs from the coding sequence of 51 individuals representing 16 monomorphic and 4 polymorphic species (Fig. 5a , Supplementary Data 1 ). Our topology was largely consistent with published phylogenies [13] , [25] , [26] , but included taxa that had not been sampled in previous phylogenies. We then phased approximately 7000 SNPs from the dsx region and built a maximum-likelihood gene tree for 116 individuals (Supplementary Data 1 ). The dsx gene tree topology mirrored the species tree topology, with the polymorphic haplotypes clustering by species (Fig. 5b ). We observed no clustering of haplotypes between species indicative of dsx allele sharing. Fig. 5: Phylogenetic relationships and evolution of mimicry in Papilio . Maximum-likelihood phylogenies for polymorphic (red) and monomorphic (black) Papilio butterflies based on genome-wide SNPs ( a ) and phased dsx SNPs ( b ). Full size image We were surprised to find all mimicry haplotypes clustering by species in the dsx gene tree, with no apparent allele clustering between species. However, ongoing recombination or gene conversion between dsx haplotypes within species could erode signatures of allele sharing due to ancestry or hybridization. Gene conversion occurs when one allelic sequence is copied onto its homolog during DNA repair, resulting in homogenization of alleles over lengths of 100–2000 bp [27] . 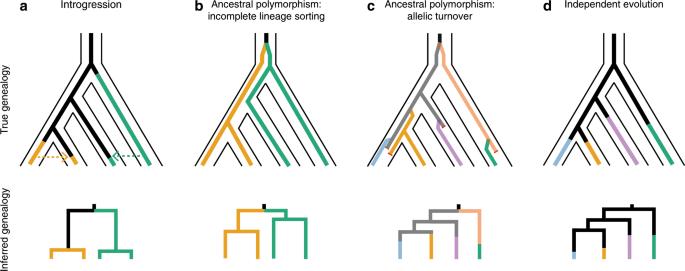Fig. 1: True (top row) and inferred (bottom row) genealogies under four mimicry evolution hypotheses. Colors represent distinct mimicry alleles/phenotypes.aMimicry alleles are shared because of introgressive hybridization.bMimicry evolves ancestrally, and descendant lineages inherit and maintain the ancestral alleles.cMimicry evolves ancestrally, and alleles are gained and lost so that the extant alleles are distinct from the ancestral alleles.dUnique mimicry alleles arise by the independent evolution of mimicry. Under introgression and incomplete lineage sorting (ILS), the inferred genealogies will show alleles grouping by phenotype rather than species (a,b), but the branch lengths will be relatively shorter for introgression than for ILS. Under allelic turnover and independent evolution, the inferred genealogies will result in alleles grouping by species (c,d), but the branch lengths are expected to be longer for allelic turnover because of underlying balancing selection. A history of allelic turnover will also leave behind population genetic signatures of balancing selection, such as elevated Tajima’s D in the region of interest. Under allelic turnover, the amount of shared ancestral variation should track phylogenetic relatedness, because recombination and gene conversion will erase the evidence of ancestral variants as a lineage ages. Because shared ancestral variation is more likely to be retained at younger timescales, allelic genealogies may show alleles of one species nested within another species for younger lineages. In contrast, independent evolution need not involve balancing selection, and if variants are shared among lineages, these should not be correlated with the lineages’ phylogenetic proximity. We tested for gene conversion between dsx haplotypes within each polymorphic species using GENECONV [28] and found two significant tracts of identical sequence (Supplementary Table 1 ). The first was in P. polytes , and coincided with a region of decreased F ST (Supplementary Table 1 , Fig. 3a ). The second putative gene conversion tract was between the P. rumanzovia simple and white morphs, and also coincided with the low F ST and LD signatures observed for that part of the dsx region (Supplementary Table 1 , Fig. 3g , Fig. 4b ). However, given the extended lengths of these putative tracts compared to typical gene conversion events, these regions appear to reflect areas of recombination between dsx alleles. While our phylogenetic analysis showed that dsx haplotypes were not shared among species, we could expect to find some trans-species polymorphisms associated with wing patterning across species if dsx haplotypes were inherited from a polymorphic ancestor. We identified SNPs associated with wing patterning in each polymorphic species, and then compared these across all species to assess if any SNPs were shared among taxa. There were some shared SNPs among species, but the number was small (1–19 SNPs), and we observed that only some combinations of species shared associated polymorphisms (5/11 comparisons; Fig. 6a ). The number of shared SNPs was higher in more phylogenetic proximate taxa, with P. rumanzovia and P. memnon sharing the most variants (Fig. 6a ). As expected, there were virtually no SNPs associated with wing pattern in the respective gene conversion/recombination tracts of P. polytes and P. rumanzovia , and therefore no shared SNPs within these regions. This suggests that any ancestrally shared variants in these regions would have been eroded away by gene conversion and recombination, thus erasing the expected phylogenetic signature of ancestral polymorphism. Fig. 6: Trans-species polymorphisms and evidence of balancing selection at dsx . a Unique and shared SNPs across the dsx (gray box) region. Vertical boxes E1–6 indicate the dsx exons. Color variation in dots is due to overlapping points. Species combinations not shown had no shared SNPs. b Genome-wide Tajima’s D distributions. Red arrows indicate the highest Tajima’s D value for dsx windows. Full size image To further explore the scenario of ancestral polymorphism, we calculated Tajima’s D for dsx -specific variants and compared these to the genome-wide distribution of Tajima’s D values for each polymorphic lineage. In each species, Tajima’s D was elevated for dsx variants (Fig. 6b ). Peak Tajima’s D values for the dsx region were in the 96 th percentile for P. polytes , the 87 th for P. rumanzovia , the 99 th for P. memnon , and the 91 st for P. aegeus . Our study reveals a dynamic history of mimicry and wing pattern evolution within Papilio that involves changes at a single autosomal gene, dsx . Although we find the same gene underlying polymorphic mimicry in multiple taxa, our analyses reveal species-specific patterns of genetic variation and linkage disequilibrium between dsx mimicry alleles. In P. polytes the mimetic and non-mimetic dsx haplotypes differ by thousands of substitutions in their coding and non-coding sequence, and an inversion spans the entire dsx gene, possibly affecting neighboring gene function [11] , [17] , [26] . In contrast, P. rumanzovia showed an extended region of genetic differentiation and LD across dsx exons two through six, but only distinguishing the white morph from the simple and blended morphs. Exon one, which codes for most of the Dsx protein and an essential DNA binding domain, is not differentiated between morphs. Furthermore, we found that the differences in dsx sequence were almost exclusively in the non-coding regions of the gene. Together these patterns suggest that variation in dsx regulation controls mimicry in P. rumanzovia , echoing previous work suggesting that dsx coding differences do not contribute to mimicry in P. polytes [26] . In P. memnon we observed signatures more similar to P. polytes , including sequence differences and high LD between morphs across the entirety of dsx and substitutions in both coding and non-coding sequence. Finally, in P. aegeus we observed differentiation between morphs in coding and non-coding sequence and high LD concentrated around exon one. While we cannot pinpoint the mutations that drive female development into alternative morphs, these results suggest that there is not a shared functional mechanism underlying dsx -mediated mimicry in different Papilio species. Recombination between dsx alleles is reduced to some degree in each polymorphic species, but reduced recombination appears to be caused by different mechanisms. In contrast to the chromosomal inversion spanning dsx in P. polytes , Iijima et al. [19] found no rearrangement between the P. memnon dsx alleles. Instead, they suggest that large indels and repetitive sequences are responsible for suppressing recombination between dsx alleles in P. memnon . Our de novo assembly similarly indicated that the P. polytes inversion breakpoints were not present in P. rumanzovia , although there still exists the possibility that a smaller inversion could be contained within the dsx region. The dsx inversion may thus be a feature specific to the P. polytes lineage. Convergent dsx -mediated mimicry could arise by different evolutionary processes including introgression, incomplete lineage sorting, allelic turnover, and/or independent evolution (Fig. 1 ). We found that dsx mimicry haplotypes are unique among taxa, inconsistent with the expected signatures of introgression or incomplete lineage sorting. While the expected signatures of introgression and incomplete lineage sorting involve clear discrepancies between gene and species trees, the scenarios of allelic turnover and independent evolution are more difficult to distinguish from one another. Allelic turnover is another outcome of ancestral polymorphism, but involves a variety of processes that result in distinct ancestral and extant alleles. Takahata [20] described this scenario in the context of the major histocompatibility complex, in which polymorphic alleles of different functional classes (analogous to wing pattern haplotypes in our system) are shared among species and maintained by balancing selection, or lost by genetic drift. In an allelic turnover event, an existing allele mutates to a new descendant allele, which then randomly replaces an existing allele. Thus, new alleles are continuously produced, and eventually replace the ancestral alleles. Adding recombination to this model effectively amplifies the effects of allelic turnover, as nucleotides are shuffled among existing alleles [29] . Allelic turnover and recombination/gene conversion will thus progressively erode trans-species polymorphisms that may have been present in the past. While aspects of the allelic turnover model are similar to normal molecular divergence, there are some clear distinctions that suggest dsx is likely evolving according to the allelic turnover model in Papilio . For instance, both allelic turnover and normal molecular divergence are expected to result in an allelic genealogy structure that matches the basic coalescent [20] , [22] . However, because allelic turnover is the product of multiallelic balancing selection, the timescale of the coalescent is expected to be different, leading to an elongation of the allelic genealogy and long terminal branches in particular [22] , [23] . Consistent with these predictions, we found that the structure of the dsx tree largely matched the genome-wide tree but the branch lengths appeared to be longer (Fig. 5 ). There were also two instances in the dsx tree in which haplotypes from one species were nested within another species ( P. ambrax within P. polytes and P. polymnestor within P. memnon , Fig. 5b ), suggesting some retention of ancestral variation at younger time scales, as expected under the allelic turnover model. Furthermore, the elevated Tajima’s D statistic in the dsx region of each polymorphic lineage is also consistent with balancing selection. Previous research has also shown this turnover process play out on relatively short timescales. Zhang et al. [26] showed that new mimicry alleles arose independently in each of two P. polytes subspecies in the course of approximately 1.7 MY, illustrating the rapid timescale of dsx turnover. They also revealed the loss of dsx polymorphism in P. ambrax and P. phestus , close relatives of P. polytes that fixed the mimetic allele and lost the non-mimetic allele due to drift and selection. These examples illustrate the gain and loss of dsx alleles in the P. polytes species group. Although we observed phylogenetically distinct dsx haplotypes among species which could have arisen by independent evolution in each lineage, we also identified several trans-species dsx polymorphisms associated with wing patterning which may further indicate that this variation predates the origin of our focal taxa. If these shared polymorphisms are indeed the remnants of an ancestral dsx wing pattern polymorphism, the evidence of ongoing gene conversion and/or recombination between dsx haplotypes helps explain why there remains little shared variation and thus the haplotypes appear to be distinct between species. Among our comparisons, P. memnon and P. rumanzovia shared the most SNPs associated with wing pattern, and are also the two most closely related polymorphic species of the four. Comparisons involving P. memnon / P. rumanzovia , and P. polytes had the second highest number of shared polymorphisms. P. aegeus , the most distant relative of the other three, only shared one associated SNP with P. polytes (and zero with P. memnon or P. rumanzovia ). This phylogenetic signal among the trans-specific polymorphism data, in which more closely related species share more wing pattern-associated variants, is consistent with the idea that these SNPs represent ancestral polymorphisms rather than being the product of recurrent mutation. Overall, our results are consistent with the predicted effects of allelic turnover and recombination/gene conversion on ancestral polymorphisms. Our findings thus indicate that the gain and loss of mimicry alleles may be widespread in shaping Papilio wing pattern diversity. Although previously regarded as an evolutionary dead-end [12] , [13] , [30] , mimicry in Papilio butterflies appears to be an ancient adaptation that has fueled the dynamic evolutionary turnover of wing patterning alleles. Sample preparation and sequencing 130 adult butterflies were collected from the wild and from butterfly farms (Supplementary Data 1 ). Approximately 10 mg of thoracic tissue was removed from each individual and genomic DNA was extracted using a chloroform-based protocol. 100 bp paired-end libraries were prepared using the KAPA Hyper Prep Kit. P. rumanzovia libraries were sequenced on an Illumina HiSeq2500 and all others were sequenced on an Illumina HiSeq4000. Raw reads were demultiplexed based on their barcodes (Supplementary Data 1 ). Data collection and genotype calling We chose to use the monomorphic outgroup species P. xuthus as the reference genome for all read-mapping instead of the more closely related P. polytes to avoid biasing our results with a polymorphic reference. We downloaded the P. xuthus v1.0 genome from PapilioBase [17] and P. polytes resequencing data from three homozygous mimetic and three homozygous non-mimetic females from NCBI (SRR1118152, SRR1118150, SRR1118145, SRR1112619, SRR1112070, SRR1111718) [11] . Reads from the 136 total genome resequencing datasets were quality trimmed using SLIDINGWINDOW:4:15 in Trimmomatic [31] and remaining reads were mapped to the P. xuthus v1.0 genome using the --very-sensitive-local option in Bowtie2 [32] . Mapped reads were then re-ordered, sorted, and deduplicated with Picard ( http://picard.sourceforge.net ). We called variants using GATK’s [33] HaplotypeCaller with options --emitRefConfidence GVCF --heterozygosity 0.01 -stand_call_conf 50.0 and performed joint genotyping using GenotypeGVCFs. For SNPs we filtered out the bottom 10% by quality and with FS > 60.0 and ReadPosRankSum λ−8.0, and for indels we filtered out the bottom 10% by quality and with FS > 200.0 and ReadPosRankSum <−20.0 using GATK’s VariantFiltration. We became aware of the presence of microsporidian sequences (specifically of Nosema bombycis ) in the P. xuthus genome assembly. We analyzed four representative datasets to verify that our results were not impacted by the presence of these sequences (see Supplementary Note 1 ). Genome-wide association and principal component analyses VCF files containing SNP and indel calls were converted to PLINK format using VCFTools [34] . Phenotypes were assigned using a custom script and files were converted to GEMMA input using PLINK [35] . We used GEMMA [36] to perform association tests between genotypes and wing pattern phenotype using option -miss 0.20. Benjamini-Hochberg false discovery rate ( q -value) [37] cutoffs of 0.01 and 0.001 were calculated for each GWAS in R [38] and manhattan plots were generated using the qqman R package [38] , [39] . We used PLINK [35] to perform PCA using only SNP calls and option --geno 0.1. PCA plots were generated using the ggplot2 package in R [38] , [40] . F ST analysis We calculated Weir and Cockerham’s F ST [41] in 10 kb windows across the genome based on SNP calls using VCFTools [34] with options --weir-fst-pop and --fst-window-size 10000. We calculated the distribution of the number of variants per window for each pairwise comparison and removed windows in the bottom 10% because these windows are more likely to show artificially extreme F ST values. F ST line graphs and distributions were plotted with the ggplot2 R package [38] , [40] . Linkage disequilibrium (LD) analysis VCF files containing SNP calls across dsx and the flanking 100 kb were converted to Haploview format using PLINK [35] . A random subset of biallelic variants was selected using PLINK’s --thin option to yield ~1000 representative variants per species. We used Haploview [42] to calculate pairwise LD between variants with a minimum genotyping rate of 75% and minimum minor allele frequency of 0.001. LD heat maps were exported from Haploview. De novo genome assembly We used genomic DNA extracted for paired-end sequencing to generate mate-pair libraries for two P. rumanzovia samples: one homozygous simple morph female and one homozygous white morph female. We size-selected DNA using the BluePippin platform (Sage Science) and constructed 3 kb mate-pair libraries using the Nextera Mate Pair Library Prep Kit (Illumina). We assembled the combined dataset of 100 bp paired-end and 3 kb mate-pair libraries for each individual using Platanus [43] . With each assembly, we then used BLAST [44] and BLAT [45] to find scaffolds containing dsx exons, using the P. polytes dsx exons as the queries. Once we had identified the relevant scaffolds we aligned them using MAFFT [46] and calculated sequence identity between the aligned regions with sliding 100 bp windows in Geneious [47] . 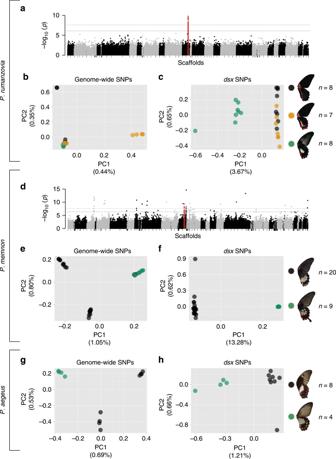Fig. 2: Identifying mimicry loci inP. rumanzovia,P. memnon, andP. aegeus. Genome-wide association study (GWAS) for wing patterning inP. rumanzovia(a) andP. memnon(d). Principal component analysis (PCA) based on genome-wide variants forP. rumanzovia(b),P. memnon(e), andP. aegeus(g). PCA based ondsxvariants forP. rumanzovia(c),P. memnon(f), andP. aegeus(h). Red points inaanddindicate SNPs in thedsxregion. Dashed and dotted lines inaanddshow the false discovery rate (q-value) cutoffs of 0.01 and 0.001, respectively. Genome-wide and dsx phylogeny estimation Approximately 3.4 million SNP calls from genome-wide coding sequence for 50 high quality individuals representing 4 polymorphic species and 16 monomorphic species were aligned in Geneious [47] and converted to PHYLIP format. We inferred a genome-wide maximum-likelihood tree using the GTRGAMMA model with 100 bootstraps in RAxML [48] . The RAxML output was uploaded to iTOL [49] to create the tree image. We phased 6730 SNPs from the dsx region for 116 individuals representing 4 polymorphic species and 16 monomorphic species using BEAGLE [50] . We aligned sequences and converted them to PHYLIP format in Geneious [47] and constructed a maximum-likelihood trees with RAxML [48] using the GRTGAMMA model and 100 bootstraps. We constructed the tree images by uploading the RAxML outputs to iTOL [49] . Gene conversion analysis We used GENECONV [28] software to test for gene conversion between dsx haplotypes. GENECONV searches for tracts of shared sequence bounded by variable sites between alleles. The software then assesses significance using permutation testing and corrects significance values for multiple comparisons and sequence length. 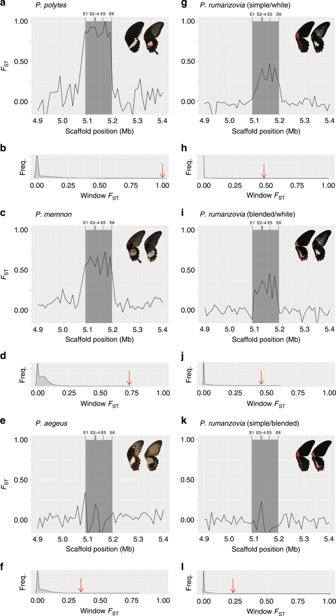Fig. 3: Genetic differentiation between morphs. FSTacross a 500 kb interval containingdsx(gray box) inP. polytes(a),P. memnon(c),P. aegeus(e), andP. rumanzovia(g,i,k). E1–6 indicate the position ofdsxexons. Genome-wideFSTdistribution inP. polytes(b),P. memnon(d),P. aegeus(f), andP. rumanzovia(h,j,l). Red arrows indicate the highestFSTvalue fordsxwindows, all of which are in the 99th percentile of their respective distributions. We used a phased full dsx region alignment (~100 kb) of all the dsx haplotypes from the polymorphic taxa as input and options -Seqtype=SILENT to minimize false positives [51] , [52] . Trans-species SNP analysis For each species, SNP calls for the dsx region were extracted and filtered using VCFTools [34] option --max-missing 0.75 to include sites were at least 75% of the individuals were genotyped. The filtered SNPs were then manually scored for genotype-wing pattern phenotype associations for each species. 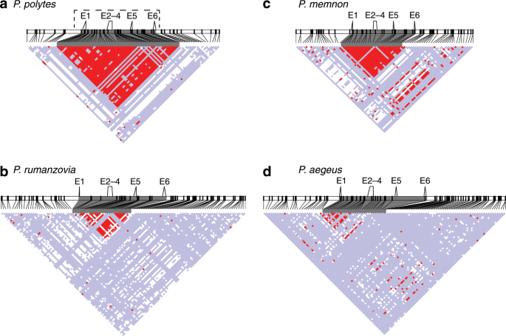Fig. 4: Linkage disequilibrium (LD) heat maps. LD acrossdsx(gray shading) and flanking 100 kb forP. polytes(a),P. rumanzovia(b),P. memnon(c), andP. aegeus(d). Standard color scheme: D’ < 1, LOD < 2 (white); D’ = 1, LOD < 2 (blue); D’ ≤ 1, LOD ≥ 2 (pink and red). Dashed line inashows the inverted region. E1–6 indicate thedsxexons. Then, R [33] was used to identify shared SNPs among species. Tajima’s D analysis For each species, we calculated Tajima’s D in 10 kb windows across the genome based on SNP calls using VCFTools [34] with option --TajimaD 10000. We calculated the distribution of the number of variants per window for each taxon and removed windows in the bottom 10%. Genome-wide Tajima’s D distributions were plotted with the ggplot2 R package [38] , [40] . 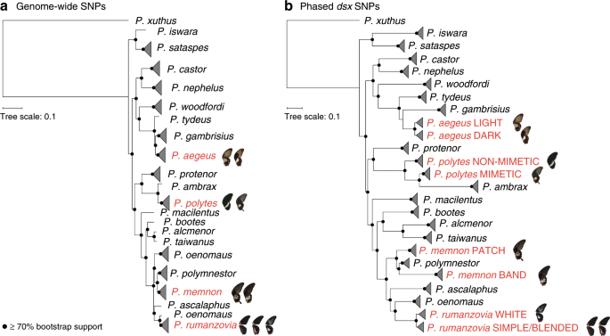Fig. 5: Phylogenetic relationships and evolution of mimicry inPapilio. Maximum-likelihood phylogenies for polymorphic (red) and monomorphic (black)Papiliobutterflies based on genome-wide SNPs (a) and phaseddsxSNPs (b). 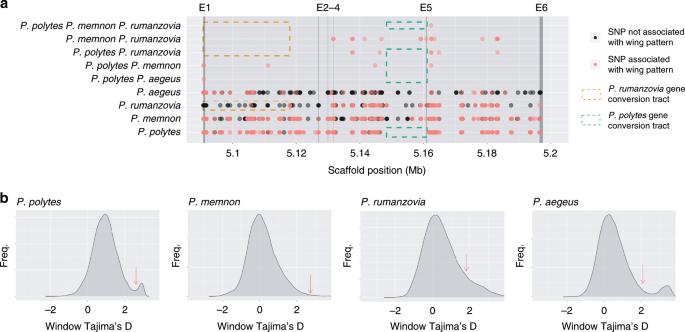Fig. 6: Trans-species polymorphisms and evidence of balancing selection atdsx. aUnique and shared SNPs across thedsx(gray box) region. Vertical boxes E1–6 indicate thedsxexons. Color variation in dots is due to overlapping points. Species combinations not shown had no shared SNPs.bGenome-wide Tajima’s D distributions. Red arrows indicate the highest Tajima’s D value fordsxwindows. Reporting summary Further information on research design is available in the Nature Research Reporting Summary linked to this article.